Iron catalysed direct alkylation of amines with alcohols The selective conversion of carbon–oxygen bonds into carbon–nitrogen bonds to form amines is one of the most important chemical transformations for the production of bulk and fine chemicals and pharma intermediates. An attractive atom-economic way of carrying out such C–N bond formations is the direct N -alkylation of simple amines with alcohols by the borrowing hydrogen strategy. Recently, transition metal complexes based on precious metals have emerged as suitable catalysts for this transformation; however, the crucial change towards the use of abundant, inexpensive and environmentally friendly metals, in particular iron, has not yet been accomplished. Here we describe the homogeneous, iron-catalysed, direct alkylation of amines with alcohols. The scope of this new methodology includes the monoalkylation of anilines and benzyl amines with a wide range of alcohols, and the use of diols in the formation of five, six- and seven- membered nitrogen heterocycles, which are privileged structures in numerous pharmaceuticals. Amines are among the most valuable classes of compounds in chemistry, omnipresent in natural products, in particular alkaloids, and widely used as pharmaceuticals, agrochemicals, lubricants and surfactants [1] , [2] , [3] . Therefore the development of efficient catalytic methodologies for C–N bond formation is a paramount goal in organic chemistry [4] . One of the most important processes to make amines is the Pd-catalysed Buchwald–Hartwig amination [5] , [6] . The choice of an alcohol [4] as substrate for direct C–N bond formation is highly desirable to produce secondary and tertiary amines and N -heterocyclic compounds ( Fig. 1 ). 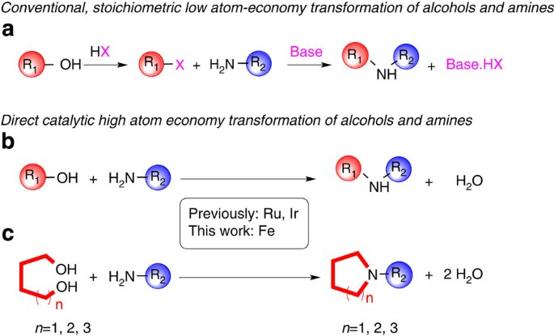Figure 1: Catalytic, directN-alkylation of amines with alcohols. (a) Conventional conversion of alcohol into amine via installing a leaving group before nucleophilic substitution with an amine donor. (b) The direct C–N bond formation via coupling of primary alcohols and amines forms secondary amine products R1–NH–R2. R1–OH is a short- or long-chain aliphatic alcohol and may contain aromatic functionality. R2–NH2is an aromatic or aliphatic amine. (c) Using diols of various chain lengths the products are 5- (n=1), 6- (n=2) or 7- (n=3) memberedN-heterocycles. Figure 1: Catalytic, direct N -alkylation of amines with alcohols. ( a ) Conventional conversion of alcohol into amine via installing a leaving group before nucleophilic substitution with an amine donor. ( b ) The direct C–N bond formation via coupling of primary alcohols and amines forms secondary amine products R 1 –NH–R 2 . R 1 –OH is a short- or long-chain aliphatic alcohol and may contain aromatic functionality. R 2 –NH 2 is an aromatic or aliphatic amine. ( c ) Using diols of various chain lengths the products are 5- ( n =1), 6- ( n =2) or 7- ( n =3) membered N -heterocycles. Full size image Alcohols are readily available through a variety of industrial processes and are highly relevant starting materials in view of recent developments in the field of renewables, as they can be obtained via fermentation or catalytic conversion of lignocellulosic biomass [7] . Conventional non-catalytic transformations of an amine with an alcohol take place via installing a suitable leaving group instead of the alcohol functionality followed by nucleophilic substitution; these multistep pathways suffer from low atom economy [8] or limited selectivity and the production of stoichiometric amounts of waste ( Fig. 1a ) [9] . A privileged catalytic methodology for the direct coupling of alcohols with amines is based on the so-called borrowing hydrogen strategy [4] ( Fig. 1b,c ). During the catalytic cycle, an alcohol is dehydrogenated to the corresponding carbonyl compound, which reacts with the amine to form an imine. The imine is in situ reduced to the alkylated amine and the metal complex facilitates the required hydrogen shuttling. In fact, the hydrogen delivered by the alcohol is temporarily stored in the metal complex. Key features are that the process is hydrogen neutral, no other reagents are needed and the only stoichiometric by-product is water. A number of transition metal complexes have proven effective in this catalytic C–N bond formation, in particular, those based on ruthenium [10] , [11] , [12] and iridium [13] . These and related methodologies have been extensively reviewed [1] , [3] , [4] , [14] , [15] , [16] . Despite recent progress, the key challenge is the development of catalysts that rely on the use of widely abundant, inexpensive metals [3] , [17] . Iron is considered to be the ultimate, sustainable alternative for ruthenium [18] ; however, no unequivocal reductive amination via a borrowing hydrogen mechanism has been reported [19] . Direct N -alkylation of amines with alcohols is limited to iron-halogenides under rather harsh reaction conditions (160–200 °C), not proceeding via a hydrogen autotransfer pathway [20] . This work shows that a well-defined homogeneous Fe-based catalyst can be successfully used in this atom-economic process, with a broad substrate scope. These direct, Fe-catalysed transformations are highly modular, and provide water, as the only stoichiometric byproduct. The products are valuable secondary and tertiary amines or heterocycles, which contain diverse moieties R 1 (from the alcohol substrate) and R 2 (from the amine substrate) ( Fig. 1 ). The presented direct waste-free alcohol to amine functional group interconversions are important toward the development of sustainable Fe-based catalysis and will enable the valorization of biomass-derived alcohols in green reaction media. Reaction design We reasoned that direct C–N bond formation with an Fe-catalyst is possible, provided the catalytic complex is bifunctional in nature and shows high activity both in alcohol dehydrogenation ( Fig. 2a , Step 1) and imine hydrogenation ( Fig. 2a , Step 3). The realization of this concept for direct alkylation of amines with alcohols using iron catalyst Cat1 ( Fig. 2b ) is presented here. Iron cyclopentadienone complex Cat1 (refs 21 , 22 , 23 ) ( Fig. 2b ) has been recently used in C=O transfer hydrogenation [24] , [25] as well as cooperative dual catalysis involving hydrogen autotransfer processes [26] . Given its unique reactivity, we considered Cat1 to be a promising candidate for the development of the desired iron-catalyzed hydrogen borrowing methodology. To achieve the direct amination of alcohols, the key challenge is to match alcohol dehydrogenation and imine hydrogenation steps by establishing conditions under which the formed Fe-H species ( Cat1-H ) from the initial alcohol dehydrogenation step is able to reduce the imine at a sufficient rate, not requiring the use of hydrogen gas. 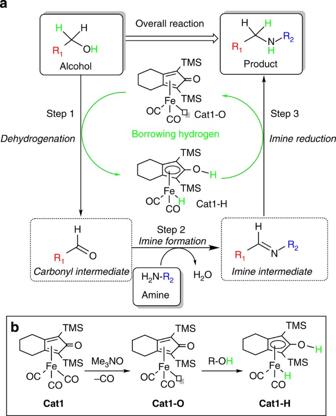Figure 2: Individual reaction steps in the iron-catalyzedN-alkylation of amines using iron cyclopentadienone complexes. (a) The overall transformation is the direct coupling of an alcohol (R1–OH) with an amine (R2–NH2) to form the product amine (R1–NH–R2). The sequence of reaction steps starts with the dehydrogenation of R1–OH to the corresponding aldehyde with iron complexCat1-O(Step 1). Thereby one ‘hydrogen equivalent’ is temporarily stored at the bifunctional iron complexCat1-O, which is converted to its reduced, hydride formCat1-H. In Step 2, the carbonyl intermediate reacts with amine R2–NH2to form an imine intermediate and water. In Step 3, the hydrogen equivalents ‘borrowed’ from alcohol R1–OH are used in the reduction of the imine intermediate to obtain the desired product R1–NH–R2. The reduction is accompanied by conversion of iron hydrideCat1-HtoCat1-O, thereby a vacant coordination site is regenerated and the catalytic cycle closed. (b) Reactivity of Fe cyclopentadienone complexes:Cat1is an air- and moisture-stable Fe-tricarbonyl precatalyst. The activeCat1-Ocomplex isin situgenerated fromCat1by the addition of 10 mol% oxidant to remove one CO.Cat1-Ois readily converted toCat1-Hby reaction with an alcohol. Figure 2: Individual reaction steps in the iron-catalyzed N -alkylation of amines using iron cyclopentadienone complexes. ( a ) The overall transformation is the direct coupling of an alcohol (R 1 –OH) with an amine (R 2 –NH 2 ) to form the product amine (R 1 –NH–R 2 ). The sequence of reaction steps starts with the dehydrogenation of R 1 –OH to the corresponding aldehyde with iron complex Cat1-O (Step 1). Thereby one ‘hydrogen equivalent’ is temporarily stored at the bifunctional iron complex Cat1-O , which is converted to its reduced, hydride form Cat1-H . In Step 2, the carbonyl intermediate reacts with amine R 2 –NH 2 to form an imine intermediate and water. In Step 3, the hydrogen equivalents ‘borrowed’ from alcohol R 1 –OH are used in the reduction of the imine intermediate to obtain the desired product R 1 –NH–R 2 . The reduction is accompanied by conversion of iron hydride Cat1-H to Cat1-O , thereby a vacant coordination site is regenerated and the catalytic cycle closed. ( b ) Reactivity of Fe cyclopentadienone complexes: Cat1 is an air- and moisture-stable Fe-tricarbonyl precatalyst. The active Cat1-O complex is in situ generated from Cat1 by the addition of 10 mol% oxidant to remove one CO. Cat1-O is readily converted to Cat1-H by reaction with an alcohol. Full size image Catalytic N -alkylation with alcohols Preliminary experiments using 4-methoxyaniline ( 1a ) and a simple aliphatic alcohol, pentane-1-ol ( 2a ), with 5 mol% pre-catalyst Cat1 and 10 mol% Me 3 NO oxidant (to form active Cat1-O ) at 110 °C in toluene showed the formation of 4-methoxy- n -pentylaniline ( 3aa ) ( Supplementary Fig. 1 ), albeit with only 30% selectivity at 48% substrate conversion (for details of optimizations, see Supplementary Table 1 ). Although promising, the initial results using common organic solvents indicated low conversion of 1a or low selectivity towards 3aa and analysis of the reaction mixtures identified insufficient imine reduction as the key problem. We reasoned that most probably a weakly coordinating ethereal solvent is needed to stabilize the key iron intermediates to enhance the imine reduction step [27] . In addition, imine formation might be facilitated in solvents, which have limited miscibility with water. The major breakthrough came when the green solvent cyclopentyl methyl ether (CPME), one that uniquely combines such properties, was selected as reaction medium. CPME recently emerged as a low-toxicity, sustainable solvent alternative for tetrahydrofuran [28] . In CPME at 110 °C, amine 1a is alkylated with pentanol to provide 3aa in 74% selectivity at 88% conversion of 1a . Full conversion of 1a and an excellent (91%) isolated yield of 3aa were obtained at slightly higher temperature (130 °C) ( Fig. 3b , Supplementary Table 1 ). Product formation profiles ( Supplementary Fig. 2 , Supplementary Table 2 ) show that the reaction is highly selective and essentially complete within 7 h. The concentration of the imine intermediate stays constantly low, and exclusive mono- N -alkylation to 3aa with increasing 1a conversion is observed. Although multiple N -alkylation is often a notorious side reaction [1] , it should be noted that the use of 1 equivalent of alcohol 2a is sufficient to form 3aa selectively and even a larger excess (6 equivalents) of 2a did not result in further alkylation of the secondary amine product ( Supplementary Table 1 ). Next, an in situ NMR study ( Supplementary Fig. 3-Ia-IIc , see Supplementary Methods for procedure) was conducted, using d 8 toluene at 100 °C that allowed the detection of all key reaction intermediates (as depicted in Fig. 2a ), that is, pentane-1-ol ( 2a ), pentan-1-al, amine 3aa and the corresponding imine, in support of the borrowing hydrogen mechanism. 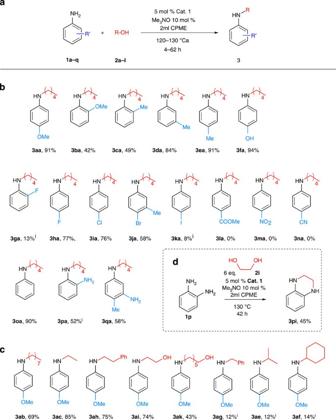Figure 3: Selective monoalkylation of functionalized anilines with various alcohols. (a) General reaction conditions. The main products areN-alkylated aniline derivatives (3). Possible side products are imines. No dialkylation is observed. (b)N-alkylation of various aniline derivatives with pentane-1-ol. Reactivity strongly depends on the substituents on the aromatic ring. Anilines bearing electron-donating groups in the para position were most reactive and3fa,3aawere obtained in 4 and 7 h, respectively.3ba,3ca,3da,3ia,3jawere obtained at prolonged reaction times at 120 °C, by addition of molecular sieves.iGC-FID selectivity is given. (c) Reactions ofp-methoxyaniline with various alcohols. Selective monoalkylation was also observed with ethane-1,2-diol and hexane-1,6-diol (3ai,3ak). (d) Direct 2,3-dihydro-quinoxaline formation from ethylene glycol ando-phenylenediamine. Figure 3: Selective monoalkylation of functionalized anilines with various alcohols. ( a ) General reaction conditions. The main products are N -alkylated aniline derivatives ( 3 ). Possible side products are imines. No dialkylation is observed. ( b ) N -alkylation of various aniline derivatives with pentane-1-ol. Reactivity strongly depends on the substituents on the aromatic ring. Anilines bearing electron-donating groups in the para position were most reactive and 3fa , 3aa were obtained in 4 and 7 h, respectively. 3ba , 3ca , 3da , 3ia , 3ja were obtained at prolonged reaction times at 120 °C, by addition of molecular sieves. i GC-FID selectivity is given. ( c ) Reactions of p -methoxyaniline with various alcohols. Selective monoalkylation was also observed with ethane-1,2-diol and hexane-1,6-diol ( 3ai , 3ak ). ( d ) Direct 2,3-dihydro-quinoxaline formation from ethylene glycol and o -phenylenediamine. Full size image Monoalkylation of various anilines with 1-pentanol The general applicability of this method for the selective monoalkylation of substituted anilines was examined using 2a and 17 different anilines 1a – 1q ( Supplementary Fig. 4 ). The isolated yields under optimized conditions are shown in Fig. 3b . The reactivity of substrates 1a – 1q was also compared under standard reaction conditions (reaction time 18 h) to assess substituent effects ( Supplementary Fig. 4 , Supplementary Table 3 ). Selective monoalkylation was observed in each case; however, the differences in reactivity were significant. Para-substituted anilines were more reactive than ortho- or meta- substituted analogues (that is, 1a versus 1b ), wheras the reactivity of toluidines increased in the order ortho ( 1c )<meta ( 1d )<para ( 1e ) probably owing to a combination of basicity and steric effects. It was furthermore established that anilines comprising electron-withdrawing substituents were less reactive and that the reactivity of para-halogenated anilines decreased in the order: fluoro ( 1 h )>chloro ( 1i )~bromo ( 1j )>iodo ( 1k ). Accordingly, the best result was obtained with p -hydroxyaniline, which was converted to 3fa in excellent 94% isolated yield already after 4 h. This increased reactivity might be attributed to the enhanced nucleophilicity of 1f or the presence of the relatively acidic phenol moiety, which likely catalyses the imine formation step. 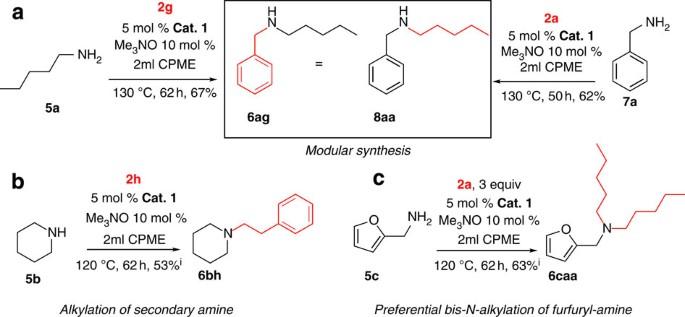Figure 4:N-Alkylation of aliphatic amines with aliphatic alcohols. (a) Modular synthesis with aliphatic amines and alcohols. Pentyl-1-amine (5a) can be coupled with benzyl-alcohol (2g) or benzyl amine (7a) is coupled with pentane-1-ol (2a) to afford the same amine product. (b) The methodology can be extended tosecondary amines, piperidine (5b) is alkylated with 2-phenyl-1-ethanol (2h). (c) The reaction of furfuryl-amine (5c) with pentane-1-ol (2a) results in bis-N-alkylation product6caa.iMolecular sieves were used. p -methoxyaniline was converted to 3aa within 7 h, and para-methylaniline ( 1e ), being less reactive, gave 3ea in 91% isolated yield after 22 h. Other substrates required further optimization, which was initially conducted using one of the least reactive substrates, 1b ( Supplementary Table 4 ). It was shown that prolonged reaction times and the addition of molecular sieves (to accelerate the imine formation step) lead to satisfactory results and products 3ba , as well as 3ca , 3da , 3ia , 3ja were isolated in moderate-to-high yields (42–84%). 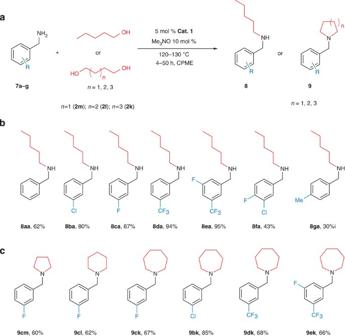Figure 5: Reactions of various benzylamines with pentane-1-ol and diols. (a) General reaction conditions. (b) Reactions of various benzyl-amines with pentanol. Benzyl-amines bearing electron-withdrawing substituents in the meta position were highly reactive, for example, for8ca,8daand8ea, no dialkylated amine or imine were observed. Benzyl amines7aand7gwere less reactive, with these substrates small amounts of dialkylated and imine products were also observed. (c) Construction of 5-, 6- or 7-memberedN-heterocyclic rings using benzylamines7b,7c,7dand7eand butane-1,4-diol (2m), pentane-1,5-diol (2l) or hexane-1,6-diol (2k). Using more reactive anilines, prolonged reaction times without the addition of molecular sieves were sufficient to obtain products 3ea , 3ha , 3oa in excellent yields (77–91%) ( Supplementary Table 5 ). Taking advantage of the distinct difference in reactivity between substituted anilines, the selective monoalkylation of 1-methyl-2,4-diamino-benzene ( 1q ) resulted in preferential formation of 3qa in 58% isolated yield. Monoalkylation of p -methoxyaniline with various alcohols Having established the reactivity pattern of anilines, we found that the selective monoalkylation of p -methoxyaniline ( 1a ) proceeds with a variety of alcohols ( 2b-2l ) with excellent results ( Fig. 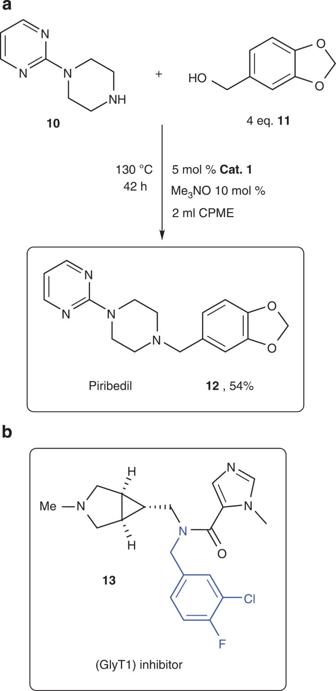Figure 6: Synthesis of pharmaceutically active molecules. (a) Iron-catalyzed direct coupling of commercially available piperazine10and piperonyl alcohol11results in the formation of Piribedil, an anti-Parkinson drug. (b) Glycine transporter type 1 (GlyT1) inhibitor, which has shown potential in the treatment of schizophrenia, containing a F-substituted benzyl-amine moiety. 3c , Supplementary Table 6 and Supplementary Figs 5 and 6 ). For instance, octanol ( 2b) , ethanol ( 2c) as well as 2-phenyl-ethane-1-ol ( 2h ) were readily converted to the corresponding amines 3ab , 3ac and 3ah in 69–85% isolated yields. Alkylations using methanol were not successful. Interestingly, selective mono-alkylation with ethane-1,2-diol ( 2i) and hexane-1,6-diol ( 2k ) delivered valuable amino-alcohols 3ai (74%) and 3ak (43%). Notably, 2,3-dihydro-quinoxaline ( 3pi ) containing a heterocyclic structure could also be constructed directly from inexpensive ethylene glycol ( Fig. 3d ). N -alkylation of aliphatic amines with aliphatic alcohols It is important that aliphatic amines can also be successfully used as reaction partners with various alcohols ( Fig. 4 , Supplementary Fig. 7 and Supplementary Table 7 ). For instance, pentane-1-amine ( 5a) was alkylated with benzylalcohol ( 2g ), providing 6ag in 67% yield. The same monoalkylated amine is obtained in 62% yield by a reverse route from benzylamine ( 7a ) and pentane-1-ol ( 2a ), showing the flexibility and versatility of the new catalytic transformation. The reaction of piperidine ( 5b ) with 2-phenyl-ethylamine ( 2h ) afforded tertiary amine 6bh in 53% isolated yield. Interestingly, furfuryl-amine ( 5c ), which can be derived from lignocellulosic biomass through furfural, displayed an interesting reactivity towards bis- N -alkylation. In the reaction of 5c with 3 equivalents of 2a , preferentially the corresponding tertiary amine ( 6caa ) was formed. Figure 4: N -Alkylation of aliphatic amines with aliphatic alcohols. ( a ) Modular synthesis with aliphatic amines and alcohols. Pentyl-1-amine ( 5a ) can be coupled with benzyl-alcohol ( 2g ) or benzyl amine ( 7a ) is coupled with pentane-1-ol ( 2a ) to afford the same amine product. ( b ) The methodology can be extended to s econdary amines, piperidine ( 5b ) is alkylated with 2-phenyl-1-ethanol ( 2h ). ( c ) The reaction of furfuryl-amine ( 5c ) with pentane-1-ol ( 2a ) results in bis- N -alkylation product 6caa . i Molecular sieves were used. Full size image N -alkylation of benzylamines N -alkylated benzyl amines are particularly important targets, as these moieties are present in a variety of drug molecules, for example, a glycine transporter type 1 inhibitor, which has shown potential in the treatment of schizophrenia [29] ( Fig. 6b ). Figure 6: Synthesis of pharmaceutically active molecules. ( a ) Iron-catalyzed direct coupling of commercially available piperazine 10 and piperonyl alcohol 11 results in the formation of Piribedil, an anti-Parkinson drug. ( b ) Glycine transporter type 1 (GlyT1) inhibitor, which has shown potential in the treatment of schizophrenia, containing a F-substituted benzyl-amine moiety. Full size image Again a distinct substituent effect was observed in the benzylamine reaction partner ( Fig. 5a,b ). Para-methyl substituted 7g and unsubstituted 7a showed lower reactivity than meta-halogen substituted benzyl amines (7 b – 7f) , which reacted much faster with pentane-1-ol ( 2a ). This is probably due to the increased rate of reduction of the corresponding imines. The effect of the aromatic ring substituents on the reaction rate can be rationalized by double bond isomerization of the formed imines to be in conjugation with the aromatic ring. Related double bond shifts in benzyl-amine derived imines were observed with the related Ru-based Shvo catalyst [30] . Substituted N -alkylated benzylamines 8ba , 8ca, 8da and 8ea were obtained in excellent, 80–95% isolated yield ( Supplementary Fig 8 , Supplementary Table 8 ). Following the alkylation over 6 h confirmed that the reactivity of benzyl amines 7a – 7e , increases in the order 7a < 7b < 7c < 7d < 7e , reflecting the increasing electronegativity of the substituents ( Supplementary Fig. 9 ). Figure 5: Reactions of various benzylamines with pentane-1-ol and diols. ( a ) General reaction conditions. ( b ) Reactions of various benzyl-amines with pentanol. Benzyl-amines bearing electron-withdrawing substituents in the meta position were highly reactive, for example, for 8ca , 8da and 8ea , no dialkylated amine or imine were observed. Benzyl amines 7a and 7g were less reactive, with these substrates small amounts of dialkylated and imine products were also observed. ( c ) Construction of 5-, 6- or 7-membered N -heterocyclic rings using benzylamines 7b , 7c , 7d and 7e and butane-1,4-diol ( 2m ), pentane-1,5-diol ( 2l ) or hexane-1,6-diol ( 2k ). Full size image Heterocycle formation with various benzylamines and diols Building on the excellent reactivity of benzyl amines 7c – 7e , we attempted the formation of nitrogen-containing heterocycles of various sizes using diols of different chain lengths (butane-1,4-diol ( 2m ), pentane-1,5-diol ( 2l ) or hexane-1,6-diol ( 2k ) ( Fig. 5c , Supplementary Table 9 ). An additional advantage of the use of benzylamines is that the free N -heterocycles can be readily obtained by common debenzylation procedures. Despite the fact that a sequential catalytic N , N -dialkylation at the same nitrogen has to occur involving each of the hydroxyl groups of the diol, we reasoned that the first intermolecular alkylation is followed by an iminium ion-based alkylation, likely facilitated by the intramolecular nature of the second alkylation step. To our delight, pyrrolidine 9 cm , containing a key five-membered heterocycle, was obtained in 60% yield from 7c and butane-1,4-ol ( 2m ). Six-membered piperidine derivative 9cl was constructed using pentane-1,5 diol ( 2l ) and 7c . As seven-membered ring formation is generally challenging in organic synthesis, it is a notable feature of our new Fe-based catalytic procedure that various azepane type N -heterocyclic compounds were readily obtained using benzyl amines 7b – 7e and hexane-1,6-diol ( 2k ). It is remarkable that in all these reactions, full conversion and perfect product selectivity was observed. Among all derivatives, the chloro-substituted 9bk was obtained with the highest isolated yield (85%). In contrast, the reaction of unsubstituted benzylamine 7a with 2k afforded the monoalkylation product, showing that the second cyclization step was much slower in this case. These results highlight the value of this methodology in accessing biological important nitrogen heterocycles, which contain -F and -CF 3 substituents. These are frequently encountered motives in pharmaceutically active compounds ( Fig. 6 ). Synthesis of pharmaceutically relevant molecules To demonstrate the power of the new C–N bond formation, we applied the Fe-catalyzed direct amine alkylation as a key connection step in the synthesis of the N -arylpiperazine drug Piribedil ( 12 ) ( Fig. 6a ), a dopamine antagonist used in the treatment of Parkinson’s disease [11] , [31] . The application of iron-based homogeneous catalyst in the preparation of pharmaceutically active molecules is highly desired, given the limited allowed ppm levels of noble metal catalysts in the final products [29] . Taking advantage of the previously established reactivity of benzyl alcohol and piperidine in our system ( Fig. 5b ), commercially available 1-(2-pyrimidyl)-piperazine ( 10 ) and 4 equivalents of piperonyl alcohol ( 11 ) were used, providing Piribedil in 54% isolated yield. This direct, base-free catalytic coupling illustrates several advantages for drug syntheses: no auxiliary reagents are required, an iron catalyst and the green solvent CPME are used, and water is the only waste product. We have developed a versatile Fe-based catalytic approach for the direct coupling of amines and alcohols. Key elements are a single bifunctional Fe-catalyst for alcohol dehydrogenation and imine hydrogenation, and the use of green solvent CPME. The variety of primary amines and alcohols, including those derived from biomass, which can be coupled, provides an excellent basis for highly flexible methodology to synthesize a broad array of secondary amines and nitrogen heterocycles and holds promise for future application in diversity-oriented synthesis strategies. The first upscaling experiments showed that this direct N -alkylation can provide up to gram amounts of secondary amines. Mechanistic investigations are needed to elucidate the role of steric and electronic parameters in the rate-determining step, which can be both the imine formation as well as the imine reduction. For example, para-hydroxy aniline was rapidly converted within 4 h, whereas o -methoxy aniline was much less reactive. Similarly, benzyl-amines display marked reactivity difference, depending on the nature and position of the substituents at the aromatic ring. We foresee that control of the reactivity of well-defined Fe-catalysts, as shown here successfully for the borrowing hydrogen strategy in the direct alkylation of amines with alcohols, will enable the discovery of a range of other new catalyst structures and sustainable transformations, using abundant iron. Standard procedure for direct alkylation of amines An oven-dried 20-ml Schlenk tube, equipped with a stirring bar, was charged with amine (0.500 mmol, 1 equivalent), alcohol (given amount), iron complex Cat 1 (0.025 mmol, 10.5 mg), Me 3 NO (0.050 mmol, 3.75 mg) and cyclopentylmethylether (solvent, 2 ml). Solid materials were weighed into the Schlenk tube under air, and the Schlenk tube was subsequently connected to an argon line and vacuum-argon exchange was performed three times. Liquid starting materials and solvent were charged under an argon stream. The Schlenk tube was capped and the mixture was rapidly stirred at room temperature for 1 min, then was placed into a pre-heated oil bath at the appropriate temperature and stirred for a given time. The crude mixture was filtered through celite, eluted with ethyl-acetate and concentrated in vacuo . The residue was purified by flash column chromatography to provide the pure amine product. Upscaling procedure for N -alkylation of p -methoxyaniline An oven-dried 100-ml Schlenk tube, equipped with a stirring bar, was charged with p -methoxyaniline (7.40 mmol, 0.910 gram, 1 equivalent), iron complex Cat 1 (0.37 mmol, 155 mg, 0.05 equivalent) and Me 3 NO (0.74 mmol, 55.5 mg, 0.10 equivalent) under air and the Schlenk tube was subsequently connected to an argon line and vacuum-argon exchange was performed three times. Then 1-pentanol (14.8 mmol, 1.62 ml, 2 equivalent), cyclopentylmethylether (solvent, 30 ml), 3 Å molecular sieves (800 mg) were charged under an argon stream. The Schlenk tube was capped and the mixture was rapidly stirred at room temperature for 3 min, then was placed into a pre-heated oil bath at 130 °C and stirred for 18 h. After cooled down to room temperature, the crude mixture was concentrated in vacuo . The residue was purified by flash column chromatography (SiO 2 , n -pentane/EtOAc 100:0 to 95:5) to provide 1.085 gram of 4-methoxy- N -pentylaniline in 76% isolated yield. For more details on synthetic procedures, see also Supplementary Methods . For NMR analysis of the isolated products in this article, see Supplementary Methods and Supplementary Figs 10–43 . How to cite this article : Yan, T. et al . Iron catalysed direct alkylation of amines with alcohols. Nat. Commun. 5:5602 doi: 10.1038/ncomms6602 (2014).